PKM2 regulates the Warburg effect and promotes HMGB1 release in sepsis Increasing evidence suggests the important role of metabolic reprogramming in the regulation of the innate inflammatory response, but the underlying mechanism remains unclear. Here we provide evidence to support a novel role for the pyruvate kinase M2 (PKM2)-mediated Warburg effect, namely aerobic glycolysis, in the regulation of high-mobility group box 1 (HMGB1) release. PKM2 interacts with hypoxia-inducible factor 1α (HIF1α) and activates the HIF-1α-dependent transcription of enzymes necessary for aerobic glycolysis in macrophages. Knockdown of PKM2, HIF1α and glycolysis-related genes uniformly decreases lactate production and HMGB1 release. Similarly, a potential PKM2 inhibitor, shikonin, reduces serum lactate and HMGB1 levels, and protects mice from lethal endotoxemia and sepsis. Collectively, these findings shed light on a novel mechanism for metabolic control of inflammation by regulating HMGB1 release and highlight the importance of targeting aerobic glycolysis in the treatment of sepsis and other inflammatory diseases. Severe sepsis and septic shock represent a major clinical problem and are the leading causes of death in patients within intensive care units worldwide [1] . This medical problem results from an exuberant and excessive host response associated with a deleterious and non-resolving systemic inflammatory response syndrome, often caused by Gram-negative bacterial infection [2] . As the major component of Gram-negative bacteria, lipopolysaccharide (LPS) can induce the secretion and release of multiple proinflammatory cytokines such as tumour necrosis factor-α (TNF-α) [3] , interleukin-1β (IL-1β) [4] and high-mobility group box 1 (HMGB1) [5] . In contrast to early proinflammatory cytokines (for example, TNF-α and IL-1β), HMGB1 is released in a delayed manner and functions as a late mediator of lethal sepsis [5] , and thus as a therapeutic target that has a wider time window for clinical intervention [6] . In resting cells, most of the HMGB1 resides in the nucleus and functions as a DNA chaperone to regulate chromosomal structure and DNA biology [7] . When actively secreted by immune cells or passively leaked from necrotic or injured cells [5] , [8] , [9] , HMGB1 functions as a damage-associated molecular pattern to mediate innate immune responses [10] . The secretion of HMGB1 from activated immune cells is a highly regulated process involving multiple steps and mechanisms. For instance, post-transcriptional modification (for example, acetylation) in the nuclear localization signal promotes HMGB1 translocation from the nucleus to the cytoplasm [11] . Subsequently, secretory lysosome-mediated exocytosis and other unknown pathways facilitate HMGB1 release into the extracellular space [12] . Therefore, a more comprehensive understanding of the mechanisms underlying the regulation of HMGB1 release by activated immune cells may ultimately lead to better treatments for patients with various inflammation-associated diseases [13] . Metabolism includes processes in which biochemicals are degraded to produce energy (in the form of adenosine triphosphate). Intermediate metabolites may serve as signalling molecules to regulate cellular processes. This metabolism-driven reprogramming dictates the progression of many cellular functions and even cellular fate. For instance, tumour cells can strategically generate adenosine triphosphate through aerobic glycolysis (in addition to oxidative phosphorylation), even when oxygen is abundant [14] , enabling exaggerated tumour cell proliferation. This phenomenon has been termed the ‘Warburg effect’ and represents one of the key hallmarks of cancer [15] . Growing evidence suggests that activated immune cells (for example, macrophages, dendritic cells and T cells) also have the ability to switch from oxidative phosphorylation to aerobic glycolysis in a manner similar to tumour cells. This alteration may contribute to the regulation of innate immune functions [16] , [17] , [18] , [19] and represents a novel target for inflammatory diseases. One key mediator of the Warburg effect is the transcription factor hypoxia-inducible factor 1α (HIF1α), a master regulator of metabolism that is upregulated in response to low oxygen or hypoxia [20] . Remarkably, a bacterial constituent, LPS, can also induce a switch from oxidative phosphorylation to aerobic glycolysis in dendritic cells and macrophages [21] , [22] , [23] and consequently results in cell activation and release of proinflammatory cytokines, including IL-1β [21] , [22] , [23] . Although the Warburg effect similarly occurs in activated macrophages, its possible role in the regulation of HMGB1 release is unknown. In the current study, we demonstrate that pyruvate kinase M2 (PKM2), a protein kinase and transcriptional coactivator, functions as an essential mediator of aerobic glycolysis [24] and an important regulator of HMGB1 release in activated macrophages. Our findings shed light on a novel mechanism for metabolic control of inflammation by regulating HMGB1 release and highlight the possibility of targeting the switch to aerobic glycolysis in the treatment of sepsis and other inflammatory diseases. Glycolysis promotes HMGB1 release To investigate whether aerobic glycolysis plays a role in the regulation of HMGB1 release, we used a glucose analogue, 2-deoxy- D -glucose (2-DG), a widely used competitive inhibitor of the first hexokinase of the glycolytic pathway. 2-DG is phosphorylated by hexokinase to 2-DG-P, which cannot be further metabolized by phosphoglucose isomerase. 2-DG (IC50≈1 mM) significantly inhibited the LPS-induced switch from oxidative phosphorylation (as measured by oxygen consumption rate (OCR)) to glycolysis (as measured by extracellular acidification rate (ECAR)) in a concentration-dependent manner ( Fig. 1a ). In parallel, 2-DG treatment also concentration-dependently inhibited the release of early (for example, IL-1β at 2 h) and late (for example, HMGB1 at 24 h) mediators in LPS-stimulated macrophages ( Fig. 1b,c ). Several immunoregulatory cytokines such as TNF-α [5] and interferon-γ (IFN-γ) [25] can induce HMGB1 release in macrophages. Similarly, 2-DG also inhibited TNF-α and IFN-γ-induced HMGB1 release in macrophages ( Fig. 1d ), suggesting a general role for glycolysis in the regulation of HMGB1 release. Although 2-DG significantly inhibited LPS-induced upregulation of IL-1β mRNA ( Fig. 1e ), it did not affect the HMGB1 mRNA levels in response to LPS, TNF-α and IFN-γ in macrophages ( Fig. 1f ). These results are consistent with those previous reports; namely, LPS induced IL-1β release in macrophages through transcriptional-dependent mechanisms, whereas LPS induced HMGB1 release in macrophages through transcriptional-independent mechanisms [5] , [22] . Collectively, our results therefore indicate a possible role for aerobic glycolysis in the regulation of HMGB1 release through post-transcriptional mechanisms. 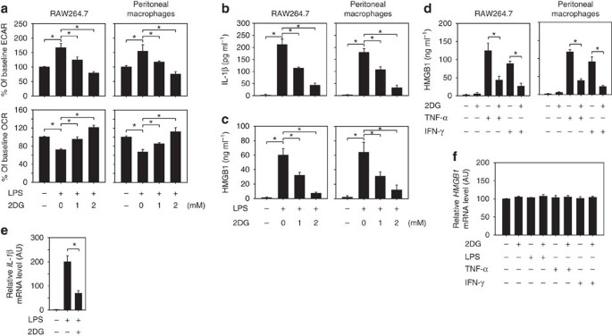Figure 1: Glycolytic inhibitor 2DG attenuates HMGB1 release by activated macrophages. (a–c) Murine RAW 264.7 macrophage cell line and primary peritoneal macrophages were pretreated with 2DG for 3 h and then stimulated with LPS (100 ng ml−1) for 2–24 h. The OCRs (indicative of oxidative phosphorylation) and ECARs (indicative of glycolysis) were monitored at 24 h using the Seahorse Bioscience Extracellular Flux Analyzer (a). The levels of secreted IL-1β at 2 h (b) and HMGB1 at 24 h (c) in the cell culture medium were measured by enzyme-linked immunosorbant assay (n=3, means±s.e.m., *P<0.05 by analysis of variance (ANOVA)LSDtest). (d) 2DG (2 mM) inhibits TNF-α (5 ng ml−1) and IFN-γ (10 ng ml−1)-induced HMGB1 release at 24 h (n=3, means±s.e.m., *P<0.05 by ANOVALSDtest). (e) IL-1β mRNA in RAW 264.7 macrophages after treatment with LPS (100 ng ml−1) for 2 h with or without 2DG (2 mM) (n=3, means±s.e.m., *P<0.05 by ANOVALSDtest). (f) HMGB1 mRNA in RAW264.7 macrophages after treatment with LPS (100 ng ml−1), TNF-α (5 ng ml−1) and IFN-γ (10 ng ml−1) for 24 h with or without 2DG (2 mM) (n=3, means±s.e.m., *P<0.05 by ANOVALSDtest). AU, arbitrary units. Figure 1: Glycolytic inhibitor 2DG attenuates HMGB1 release by activated macrophages. ( a – c ) Murine RAW 264.7 macrophage cell line and primary peritoneal macrophages were pretreated with 2DG for 3 h and then stimulated with LPS (100 ng ml −1 ) for 2–24 h. The OCRs (indicative of oxidative phosphorylation) and ECARs (indicative of glycolysis) were monitored at 24 h using the Seahorse Bioscience Extracellular Flux Analyzer ( a ). The levels of secreted IL-1β at 2 h ( b ) and HMGB1 at 24 h ( c ) in the cell culture medium were measured by enzyme-linked immunosorbant assay ( n =3, means±s.e.m., * P <0.05 by analysis of variance (ANOVA) LSD test). ( d ) 2DG (2 mM) inhibits TNF-α (5 ng ml −1 ) and IFN-γ (10 ng ml −1 )-induced HMGB1 release at 24 h ( n =3, means±s.e.m., * P <0.05 by ANOVA LSD test). ( e ) IL-1β mRNA in RAW 264.7 macrophages after treatment with LPS (100 ng ml −1 ) for 2 h with or without 2DG (2 mM) ( n =3, means±s.e.m., * P <0.05 by ANOVA LSD test). ( f ) HMGB1 mRNA in RAW264.7 macrophages after treatment with LPS (100 ng ml −1 ), TNF-α (5 ng ml −1 ) and IFN-γ (10 ng ml −1 ) for 24 h with or without 2DG (2 mM) ( n =3, means±s.e.m., * P <0.05 by ANOVA LSD test). AU, arbitrary units. Full size image PKM2 is required for active HMGB1 release The M2 isoform of PKM2 catalyses the final and rate-limiting reaction step of the glycolytic pathway and functions as the central regulator of cancer metabolism via regulating the Warburg effect [26] . However, it remains unclear whether PKM2 is also important for the Warburg effect in activated innate immune cells. Surprisingly, LPS induced a time-dependent increase in the protein and mRNA levels of PKM2 ( Fig. 2a,b ), but not PKM1 in macrophages ( Fig. 2a ), suggesting a possible role for PKM2 in the regulation of the Warburg effect as well as HMGB1 release. To test this possibility, a target-specific short hairpin RNA (shRNA) against PKM2 was transfected into RAW 264.7 macrophages. The transfection of PKM2 -shRNA led to a significant decrease in PKM2 ( Fig. 2a,b ), but not PKM1 protein levels ( Fig. 2a ). In parallel, the knockdown of PKM2 was associated with a decrease in LPS-induced glycolysis ( Fig. 2c ) and accompanying reduction of HMGB1 release ( Fig. 2d ). Treatment with a potential PKM2 inhibitor, shikonin [27] , also resulted in significant inhibition of LPS-, TNF-α- and IFN-γ-induced HMGB1 release ( Fig. 2e ). Furthermore, the knockdown of PKM2 by lentiviral shRNA in primary bone marrow macrophages (BMMs) led to inhibition of LPS-, TNF-α- and IFN-γ-induced HMGB1 release ( Fig. 2f,g ). Collectively, these results support an important role for PKM2-mediated glycolysis in the regulation of HMGB1 release in activated macrophages. 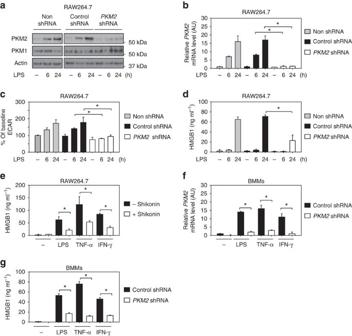Figure 2: Upregulated PKM2 promotes aerobic glycolysis and HMGB1 release in activated macrophages. (a–d) RAW 264.7 cells were transfected with or without indicated shRNA for 48 h and then stimulated with LPS (100 ng ml−1) for 6–24 h. The level of indicated protein (a), mRNA (b), ECAR (c) and HMGB1 release (d) were assayed as described in the Methods (n=3, means±s.e.m., *P<0.05 by analysis of variance (ANOVA)LSDtest). AU, arbitrary units. (e) RAW 264.7 cells were pretreated with shikonin (5 μM) for 3 h and then stimulated with LPS (100 ng ml−1), TNF-α (5 ng ml−1) and IFN-γ (10 ng ml−1) for 24 h. HMGB1 release was assayed by enzyme-linked immunosorbant assay (n=3, means±s.e.m., *P<0.05 by ANOVALSDtest). (f,g) BMMs were transfected with or without indicated shRNA for 48 h and then stimulated with LPS (100 ng ml−1), TNF-α (5 ng ml−1) and IFN-γ (10 ng ml−1) for 24 h. The mRNA levels of PKM2 (f) and HMGB1 release (g) were assayed (n=3, means±s.e.m., *P<0.05 by ANOVALSDtest). AU, arbitrary units. Figure 2: Upregulated PKM2 promotes aerobic glycolysis and HMGB1 release in activated macrophages. ( a – d ) RAW 264.7 cells were transfected with or without indicated shRNA for 48 h and then stimulated with LPS (100 ng ml −1 ) for 6–24 h. The level of indicated protein ( a ), mRNA ( b ), ECAR ( c ) and HMGB1 release ( d ) were assayed as described in the Methods ( n =3, means±s.e.m., * P <0.05 by analysis of variance (ANOVA) LSD test). AU, arbitrary units. ( e ) RAW 264.7 cells were pretreated with shikonin (5 μM) for 3 h and then stimulated with LPS (100 ng ml −1 ), TNF-α (5 ng ml −1 ) and IFN-γ (10 ng ml −1 ) for 24 h. HMGB1 release was assayed by enzyme-linked immunosorbant assay ( n =3, means±s.e.m., * P <0.05 by ANOVA LSD test). ( f , g ) BMMs were transfected with or without indicated shRNA for 48 h and then stimulated with LPS (100 ng ml −1 ), TNF-α (5 ng ml −1 ) and IFN-γ (10 ng ml −1 ) for 24 h. The mRNA levels of PKM2 ( f ) and HMGB1 release ( g ) were assayed ( n =3, means±s.e.m., * P <0.05 by ANOVA LSD test). AU, arbitrary units. Full size image PKM2-mediated HIF1α activation is required for HMGB1 release In cancer cells, PKM2 physically interacts with HIF1α in the nucleus and activates the transcription of glycolysis-related genes such as GLUT1 (glucose transporter 1, which increases glucose uptake), LDHA (lactate dehydrogenase A, which increases lactate production) and PDK1 (pyruvate dehydrogenase kinase 1, which blocks the entry of pyruvate into the tricarboxylic acid cycle) [28] . In LPS-stimulated RAW264.7 cells and primary BMMs, the interaction between PKM2 and HIF1α was markedly elevated, as determined by immunoprecipitation assays ( Fig. 3a ). However, the knockdown of PKM2 by RNA interference impaired LPS-induced HIF1α transcriptional activation ( Fig. 3b ), as well as the consequent expression of GLUT1 ( Fig. 3c ), LDHA ( Fig. 3d ) and PDK1 mRNAs ( Fig. 3e ). Notably, the knockdown of PKM2 did not affect LPS-induced HIF1α protein expression ( Fig. 3f ), suggesting an important role of PKM2-HIF1α interaction in the regulation of the transcriptional activity, but not the stability of HIF1α protein in activated macrophages. To confirm the roles of HIF1α as well as its target glycolysis-related genes in the regulation of HMGB1 release, various shRNA constructs were transfected into cultured macrophages. Interestingly, the knockdown of HIF1 α ( Fig. 3g ), GLUT1 ( Fig. 3h ), LDHA ( Fig. 3i ) and PDK1 ( Fig. 3i ) by RNA interference uniformly impaired LPS-induced HMGB1 release. Together, these findings suggest a novel role for PKM2-mediated HIF1α activation in the regulation of HMGB1 release by activated macrophages. 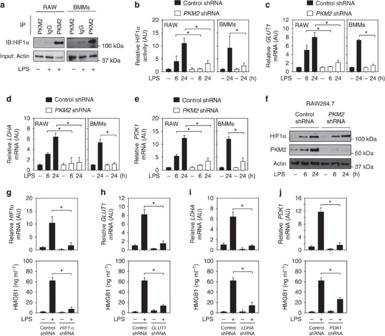Figure 3: PKM2-mediated HIF1α activation is required for HMGB1 release in activated macrophages. (a) RAW 264.7 cells (RAW) and BMMs were stimulated with LPS (100 ng ml−1) for 24 h. The interaction between PKM2 and HIF1α was assayed by immunoprecipitation (IP) and immune blotting (IB). (b–f) RAW 264.7 cells and BMMs were transfected with control shRNA or PKM2 shRNA for 48 h and then stimulated with LPS (100 ng ml−1) for 6–24 h. The mRNA levels of indicated genes (b–e) were assayed by real-time PCR (n=3, means±s.e.m., *P<0.05 by ANOVALSDtest). AU, arbitrary units. The protein level of HIF1α was assayed by western blotting (f). (g–j) RAW 264.7 cells were transfected with indicated shRNA for 48 h and then stimulated with LPS (100 ng ml−1) for 24 h. The mRNA levels of indicated genes were assayed by real-time PCR. In parallel, the extracellular levels of HMGB1 were assayed by enzyme-linked immunosorbant assay (n=3, means±s.e.m., *P<0.05 by analysis of varianceLSDtest). AU, arbitrary unit. Figure 3: PKM2-mediated HIF1α activation is required for HMGB1 release in activated macrophages. ( a ) RAW 264.7 cells (RAW) and BMMs were stimulated with LPS (100 ng ml −1 ) for 24 h. The interaction between PKM2 and HIF1α was assayed by immunoprecipitation (IP) and immune blotting (IB). ( b – f ) RAW 264.7 cells and BMMs were transfected with control shRNA or PKM2 shRNA for 48 h and then stimulated with LPS (100 ng ml −1 ) for 6–24 h. The mRNA levels of indicated genes ( b – e ) were assayed by real-time PCR ( n =3, means±s.e.m., * P <0.05 by ANOVA LSD test). AU, arbitrary units. The protein level of HIF1α was assayed by western blotting ( f ). ( g – j ) RAW 264.7 cells were transfected with indicated shRNA for 48 h and then stimulated with LPS (100 ng ml −1 ) for 24 h. The mRNA levels of indicated genes were assayed by real-time PCR. In parallel, the extracellular levels of HMGB1 were assayed by enzyme-linked immunosorbant assay ( n =3, means±s.e.m., * P <0.05 by analysis of variance LSD test). AU, arbitrary unit. Full size image Lactate promotes HMGB1 acetylation and release As the end product of glycolysis, lactate accumulated at increased levels (5–7 mM) in the culture medium of LPS-stimulated macrophages ( Fig. 4a ). In contrast, the knockdown of PKM2 and HIF1α prevented LPS-induced lactate accumulation in the culture medium ( Fig. 4a ). To understand the role of lactate in the regulation of HMGB1 release, we tested whether supplementation of exogenous lactate could induce HMGB1 release. Indeed, exposure of macrophage cultures to lactate (5 mM for 6 h) triggered a marked HMGB1 release without reducing cell viability ( Fig. 4b,c ). The recently identified lactate receptor GPR81 (ref. 29 ) was responsible for this effect ( Fig. 4b,c ). In addition, intermediate metabolites of glycolysis such as 3-phosphoglycerate, 2-phosphoglycerate and phosphoenolpyruvate (PEP) can induce lactate production and HMGB1 release in macrophages ( Fig. 4d ). Acetylation is a post-translational modification that can promote HMGB1 cytoplasmic translocation and subsequent release in response to various inflammatory stimuli as well as hypoxia [11] , [30] . Lactate increased HMGB1 acetylation ( Fig. 4e ), whereas LPS-induced HMGB1 acetylation was impaired by the knockdown of PKM2 and HIF1α ( Fig. 4f ). To gain insight into the mechanisms underlying glycolysis-mediated HMGB1 hyperacetylation, we assayed the activity of histone deacetylases (HDACs), which have been shown to acetylate both histone and non-histone nuclear proteins, including HMGB1 (refs 11 , 30 ). Similar to LPS and HDAC inhibitors (for example, trichostatin A), lactate and PEP also decreased the activity of HDACs in macrophage cultures ( Fig. 4g–j ). Collectively, these findings suggest that LPS-induced lactate production from PKM2-mediated aerobic glycolysis may act as an inhibitory signal for HDAC activity, which in turn enables HMGB1 hyperacetylation and subsequent release by LPS-stimulated macrophages. 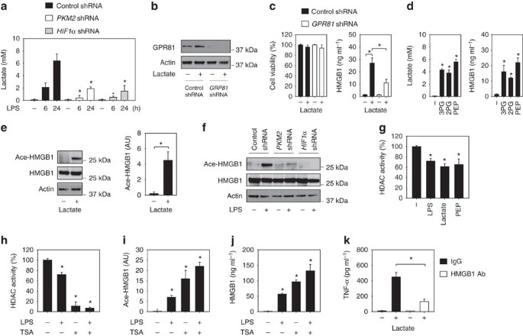Figure 4: Lactate promotes HMGB1 acetylation and release. (a) RAW 264.7 cells were transfected with indicated shRNA for 48 h and then stimulated with LPS (100 ng ml−1) for 6–24 h. The lactate level in the culture medium was assayed (n=3, means±s.e.m., *P<0.05 versus control shRNA group by analysis of variance (ANOVA)LSDtest). (b,c) RAW 264.7 cells were transfected with GRP81 shRNA and control shRNA for 48 h and then stimulated with lactate (5 mM) for 6 h. GRP81 expression (b), cell viability (c) and HMGB1 release (c) were assayed (n=3, means±s.e.m., *P<0.05 by ANOVALSDtest). (d) RAW 264.7 cells were stimulated with 3-phosphoglycerate (3PG, 2 mM), 2-phosphoglycerate (2PG, 2 mM) and PEP (2 mM) for 6 h and levels of lactate and HMGB1 release were assayed (n=3, means±s.e.m., *P<0.05 versus untreated group by ANOVALSDtest). (e) RAW 264.7 cells were stimulated with lactate (5 mM) for 6 h and levels of acetylated HMGB1 were assayed. (f) RAW 264.7 cells were stimulated with LPS (100 ng ml−1) for 24 h and the levels of acetylated HMGB1 were assayed. (g) RAW 264.7 cells were stimulated with LPS (100 ng ml−1), lactate (5 mM) and PEP (2 mM) for 24 h. HDAC activity was assayed (n=3, means±s.e.m., *P<0.05 versus untreated group by ANOVALSDtest). (h–j) RAW 264.7 cells were stimulated with Trichostatin A (TSA) (2 μM) and/or LPS (100 ng ml−1) for 24 h. HDAC activity (h) and acetylated HMGB1 (i) and HMGB1 release (j) were assayed (n=3, means±s.e.m., *P<0.05 by ANOVALSDtest). (k) RAW 264.7 cells were stimulated with lactate (5 mM, 6 h) with or without anti-HMGB1-neutralizing antibody (2 μg ml−1) and levels of TNF-α release were assayed (n=3, means±s.e.m., *P<0.05 by ANOVALSDtest). Figure 4: Lactate promotes HMGB1 acetylation and release. ( a ) RAW 264.7 cells were transfected with indicated shRNA for 48 h and then stimulated with LPS (100 ng ml −1 ) for 6–24 h. The lactate level in the culture medium was assayed ( n =3, means±s.e.m., * P <0.05 versus control shRNA group by analysis of variance (ANOVA) LSD test). ( b , c ) RAW 264.7 cells were transfected with GRP81 shRNA and control shRNA for 48 h and then stimulated with lactate (5 mM) for 6 h. GRP81 expression ( b ), cell viability ( c ) and HMGB1 release ( c ) were assayed ( n =3, means±s.e.m., * P <0.05 by ANOVA LSD test). ( d ) RAW 264.7 cells were stimulated with 3-phosphoglycerate (3PG, 2 mM), 2-phosphoglycerate (2PG, 2 mM) and PEP (2 mM) for 6 h and levels of lactate and HMGB1 release were assayed ( n =3, means±s.e.m., * P <0.05 versus untreated group by ANOVA LSD test). ( e ) RAW 264.7 cells were stimulated with lactate (5 mM) for 6 h and levels of acetylated HMGB1 were assayed. ( f ) RAW 264.7 cells were stimulated with LPS (100 ng ml −1 ) for 24 h and the levels of acetylated HMGB1 were assayed. ( g ) RAW 264.7 cells were stimulated with LPS (100 ng ml −1 ), lactate (5 mM) and PEP (2 mM) for 24 h. HDAC activity was assayed ( n =3, means±s.e.m., * P <0.05 versus untreated group by ANOVA LSD test). ( h – j ) RAW 264.7 cells were stimulated with Trichostatin A (TSA) (2 μM) and/or LPS (100 ng ml −1 ) for 24 h. HDAC activity ( h ) and acetylated HMGB1 ( i ) and HMGB1 release ( j ) were assayed ( n =3, means±s.e.m., * P <0.05 by ANOVA LSD test). ( k ) RAW 264.7 cells were stimulated with lactate (5 mM, 6 h) with or without anti-HMGB1-neutralizing antibody (2 μg ml −1 ) and levels of TNF-α release were assayed ( n =3, means±s.e.m., * P <0.05 by ANOVA LSD test). Full size image A previous study demonstrated that lactate stimulates Toll-like receptor (TLR)-4 signalling activation in macrophages [31] . In addition, HMGB1 can stimulate TNF-α release through TLR4 (ref. 32 ). We demonstrated that HMGB1-neutralizing antibody significantly inhibits lactate-induced TNF-α release ( Fig. 4k ). These findings suggest that lactate promotes macrophage activation via an autocrine HMGB1-dependent pathway. Shikonin protects mice from endotoxic shock and sepsis Given the capacity of the PKM2 inhibitor shikonin to attenuate LPS-induced IL-1β and HMGB1 release in vitro , we determined whether shikonin protects mice against lethal endotoxemia by inhibiting cytokine release. Repetitive administration of shikonin at −0.5, +12 and +24 h following the onset of endotoxemia (5 mg kg −1 LPS, intraperitoneally (i.p.)) conferred significant protection against lethal endotoxemia ( Fig. 5a ) and simultaneously reduced the PKM2 activity in peritoneal macrophages ( Fig. 5b ) and the serum levels of lactate ( Fig. 5c ), IL-1β ( Fig. 5d ) and HMGB1 ( Fig. 5e ) in endotoxemic mice. All of these mice were observed for at least 2 weeks and no late deaths occurred. These findings suggest that shikonin does not merely delay animal lethality by attenuating the production of lactate and cytokines, but also provides long-lasting protection. Although endotoxemia is a useful animal model for investigating the complex network of cytokines, a more clinically relevant experimental model for sepsis is bacterial infection induced by caecal ligation and puncture (CLP). At +24, +48 and +72 h following the onset of sepsis, animals were given shikonin or vehicle i.p. Shikonin rescued mice from CLP-induced lethal sepsis, even if given after the onset of sepsis ( Fig. 5f ). All of these mice were observed for at least 2 weeks and no late deaths occurred. The PKM2 activity in peritoneal macrophages ( Fig. 5g ) and the serum levels of lactate ( Fig. 5h ) and HMGB1 ( Fig. 5i ) were significantly decreased in the group receiving shikonin treatment for CLP. Collectively, these data suggest that the PKM2 inhibitor shikonin protects against experimental lethal endotoxic shock and sepsis partly by inhibiting PKM2 activity, lactate production and HMGB1 release. 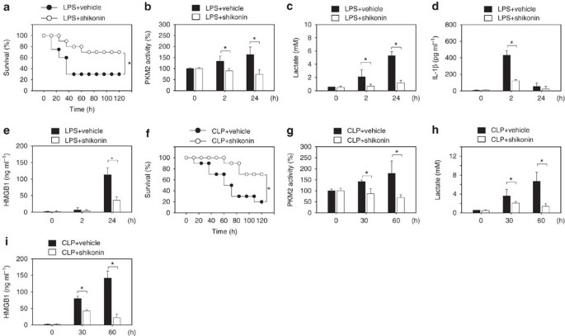Figure 5: A potential PKM2 inhibitor shikonin protects mice from lethal endotoxemia and sepsis. (a) Mice (n=20 per group) were injected with a single dose of shikonin (8 mg kg−1), followed 30 min later by an infusion of endotoxin (LPS, 5 mg kg−1, i.p.), and were then re-treated with shikonin 12 and 24 h later. The Kaplan–Meyer method was used to compare the differences in survival rates between groups (*P<0.05). (b–e) In parallel experiments, the PKM2 activity in peritoneal macrophages (b) and serum levels of lactate (c), IL-1β (d) and HMGB1 (e) at indicated time points were measured (n=3–5 animals per group, values are mean±s.e.m., *P<0.05 by analysis of variance (ANOVA)LSDtest). (f) The CLP technique was used to induce intra-abdominal sepsis in mice (n=20 per group). Repeated administration of shikonin (8 mg kg−1) at 24, 48 and 72 h after CLP significantly increased survival, as compared with vehicle group (*P<0.05), as measured by Kaplan–Meyer test. (g–i) In parallel, the PKM2 activity in peritoneal macrophages (g) and serum levels of lactate (h) and HMGB1 (i) at indicated time points were measured (n=3–5 animals per group, values are mean±s.e.m., *P<0.05 by ANOVALSDtest). Figure 5: A potential PKM2 inhibitor shikonin protects mice from lethal endotoxemia and sepsis. ( a ) Mice ( n =20 per group) were injected with a single dose of shikonin (8 mg kg −1 ), followed 30 min later by an infusion of endotoxin (LPS, 5 mg kg −1 , i.p. ), and were then re-treated with shikonin 12 and 24 h later. The Kaplan–Meyer method was used to compare the differences in survival rates between groups (* P <0.05). ( b – e ) In parallel experiments, the PKM2 activity in peritoneal macrophages ( b ) and serum levels of lactate ( c ), IL-1β ( d ) and HMGB1 ( e ) at indicated time points were measured ( n =3–5 animals per group, values are mean±s.e.m., * P <0.05 by analysis of variance (ANOVA) LSD test). ( f ) The CLP technique was used to induce intra-abdominal sepsis in mice ( n =20 per group). Repeated administration of shikonin (8 mg kg −1 ) at 24, 48 and 72 h after CLP significantly increased survival, as compared with vehicle group (* P <0.05), as measured by Kaplan–Meyer test. ( g – i ) In parallel, the PKM2 activity in peritoneal macrophages ( g ) and serum levels of lactate ( h ) and HMGB1 ( i ) at indicated time points were measured ( n =3–5 animals per group, values are mean±s.e.m., * P <0.05 by ANOVA LSD test). Full size image To ensure a timely response to infection, effective innate recognition systems that rapidly detect various microbial products such as LPS have evolved in mammals. The effective recognition of pathogen-associated molecular patterns by innate immune cells triggers the sequential release of early (for example, TNF-α and IL-1β) and late (for example, HMGB1) proinflammatory cytokines. Appropriate inflammatory responses facilitate innate immunity against infections, but excessive inflammation may also result in sepsis and even death [1] , [2] . The molecular mechanisms underlying the innate immune system response to LPS are not completely understood. In this study, we demonstrate that PKM2-mediated aerobic glycolysis contributes to macrophage activation and the resultant inflammatory response. As a co-activator, PKM2 interacts with HIF-1α and activates the transcription of glycolysis-related genes, leading to excessive lactate production and HMGB1 hyperacetylation and its subsequent release. Moreover, genetic and/or pharmacological inhibition of PKM2 significantly impairs LPS-induced HMGB1 release in macrophages and protects mice from lethal endotoxic shock and sepsis. These findings provide novel insight into the mechanisms underlying the metabolic control of inflammation and highlight the importance of targeting aerobic glycolysis in the treatment of patients with sepsis and other inflammatory diseases. The Warburg effect, first observed in various tumour cells, is also increasingly recognized as an essential regulator of innate and adaptive immunity. For instance, increased aerobic glycolysis contributes to the maturation of dendritic cells in response to TLR4, TLR2 and TLR9 ligands [21] , and influences the differentiation of both anti-inflammatory regulatory T cells and pro-inflammatory Th17 cells [33] , [34] . There are two major types of macrophages [35] : the classical M1 phenotype, which can be activated by LPS and IFN-γ to orchestrate proinflammatory responses, and the alternate M2 phenotype, which is activated by IL-4, IL-13, IL-10 and TGF-β to fulfill anti-inflammatory functions. LPS can induce the metabolic switch to aerobic glycolysis only in M1 macrophages, which contributes to transcriptional expression and release of early proinflammatory cytokines (for example, IL-1β) [22] . In this study, we found that increased aerobic glycolysis also contributes to LPS-induced release of late mediators (for example, HMGB1) by modulating its post-translational modification (rather than transcriptional expression). It now appears that the Warburg effect can participate in the regulation of proinflammatory cytokines at both the transcriptional and post-transcriptional levels. Although PKM2 is expressed at extremely low levels (if any at all) in quiescent and normally differentiated cells, its expression levels are markedly upregulated in rapidly proliferating tumour cells as well as activated macrophages. Elevated PKM2 expression in cancer cells [26] and activated immune cells enables the metabolic switch from oxidative phosphorylation to aerobic glycolysis. In cancer cells, PKM2 contributes to the Warburg effect by interacting and activating HIF-1α to induce the expression of glycolytic genes [28] . Here we demonstrate that PKM2 fulfills similar functions by interacting with HIF1α to regulate the expression of LPS-induced glycolytic genes and release of proinflammatory cytokines in macrophages. Consistently, the knockdown of PKM2 , HIF1 α, as well as aerobic glycolysis-related genes (for example, GLUT1 , LDHA and PDK1 ) significantly impaired LPS-induced HMGB1 release, suggesting an important role of the PKM2-HIF1α glycolysis pathway in the regulation of HMGB1 release by activated macrophages. Intriguingly, it has been suggested that hyperglycaemia aggravates LPS-induced HMGB1 release, whereas insulin can decrease serum HMGB1 levels in septic animals [36] , implying a possible role of glucose metabolism in the regulation of HMGB1 release. The mechanisms underlying the regulation of PKM2 expression in macrophages remains a subject of future investigation. In cancer cells, however, the expression of PKM2 is controlled by several transcription factors such as Sp1 (ref. 37 ), nuclear factor-κB [38] and Myc [39] , as well as HIF1α [28] . In addition, activation of the extracellular signal-regulated kinase is required for PKM2 expression and nuclear translocation during aerobic glycolysis [40] . Given the essential role of extracellular signal-regulated kinase in regulating active HMGB1 secretion [41] , elucidating the mechanism underlying the regulation of PKM2 upregulation in activated immune cells will be important. Hypoxia and inflammation are often intimately associated under various conditions. Hypoxia is not only a prominent feature in inflamed and injured tissues but also an effective inducer of inflammatory responses [42] , [43] . Under hypoxic conditions, HIF1α, the master regulator of the cellular response to hypoxia, can escape degradation by the ubiquitin-proteasome pathway, thereby accumulating at high levels [44] . Similarly, bacterial products (for example, LPS) [45] and proinflammatory cytokines (for example, TNF-α and IFN-γ) [46] , [47] can also stabilize HIF1α and activate relevant signalling pathways, even under normoxic conditions. In the present study, we found that knockdown of HIF1α impaired LPS-induced HMGB1 release by macrophages under normoxic conditions. Similarly, others have found that conditional knockout of HIF1α in myeloid cells (including macrophages) decreased inflammatory responses in vivo [48] and protected animals against LPS-induced lethality [49] . Activated macrophages/monocytes acetylate HMGB1 at its nuclear localization sequences, leading to sequestration of HMGB1 within cytoplasmic vesicles and subsequent release into the extracellular milieu. Extracellular HMGB1 functions as a late mediator of lethal endotoxemia and sepsis, because HMGB1-neutralizing antibodies or inhibitors reverse the course of established experimental sepsis even when these antidotes are given up to 24 h after induction of experimental sepsis [5] , [50] , [51] . These findings support the idea of HMGB1 as a promising therapeutic target to allow rescue from lethal sepsis. It is thus important to fully understand the intricate mechanisms underlying the regulation of HMGB1 release under relevant pathological conditions. Our present study reveals a crucial role for the PKM2 pathway in the regulation of HMGB1 release and suggests another possible therapeutic target for sepsis. Indeed, a potential PKM2 inhibitor [27] , shikonin, conferred significant protection against lethal endotoxemia and sepsis partly by attenuating systemic accumulation of lactate and proinflammatory cytokines. Of note, increased serum lactate levels have been suggested as a biomarker of organ failure and mortality in patients with sepsis, trauma and other critical illnesses [52] , [53] , [54] . Our findings that lactate can effectively stimulate macrophages to release HMGB1 provide a logical explanation for lactate clearance as a therapy for sepsis and other inflammatory diseases. As a component of Chinese herbal medicine, shikonin also has antioxidant properties [55] and has been tested for efficacy in the treatment of microbial infections and cancer in experimental and clinical settings [56] . It is essential to determine whether other HMGB1 inhibitors (for example, epigallocatechin gallate, tanshinone, carbenoxolone and quercetin) confer protection against lethal sepsis similarly by inhibiting the PKM2-mediated Warburg effect in innate immune cells. Collectively, our findings reveal a novel PKM2-dependent mechanism for the metabolic control of inflammation. Upregulation of PKM2 expression enables a metabolic switch to aerobic glycolysis, leading to excessive production of lactate. By inhibiting HDAC activity [57] , lactate in turn increases HMGB1 hyperacetylation, translocation to the cytoplasm and subsequent release into the extracellular milieu. Thus, novel therapeutic strategies targeting aerobic glycolysis for the treatment of patients with sepsis and other inflammatory diseases are in order. Reagents LPS ( Escherichia coli LPS 0111:B4; L4391), 2DG (D8375), trichostatin A (8552), 3-phosphoglycerate (P8877), 2-phosphoglycerate (19710) and PEP (#860077) were obtained from Sigma (St Louis, MO, USA). Shikonin (CAS 517-89-5) was obtained from EMD Millipore Corporation (Billerica, MA, USA). Mouse TNF-α (410-MT-010) and IFN-γ (485-MI-100) were obtained from R&D Systems (Minneapolis, MN, USA). Mouse anti-HMGB1 2G7 neutralizing antibody was a generous gift from Kevin J. Tracey (The Feinstein Institute for Medical Research, Manhasset, NY, USA) [32] . Cell culture Murine macrophage-like RAW 264.7 cells were obtained from the American Type Culture. Mouse peritoneal and BMMs were isolated from Balb/C mice [58] , [59] . These cells were cultured in DMEM medium (supplemented with 10% heat-inactivated fetal bovine serum and 100 units of penicillin and 100 μg ml −1 streptomycin) at 37 °C, 95% humidity and 5% CO 2 . Animal model of endotoxemia and sepsis This study was approved by the Xiangya Hospital Institutional Ethics Committee and performed in accordance with Association for Assessment and Accreditation of Laboratory Animal Care guidelines ( http://www.aaalac.org/ ). Endotoxemia was induced in Balb/C mice (male, 7–8 weeks old, 20–25 g) by i.p. injection of bacterial endotoxin (LPS, 5 mg kg −1 ) [5] , [51] . Sepsis was induced in male Balb/C mice (male, 7–8 weeks old, 20–25 g) by CLP [5] , [51] . Shikonin was dissolved in vehicle (10% dimethylsulphoxide, 20% Cremophor:ethanol (3:1) and 70% PBS) and administered i.p. to mice at the indicated time points. Blood was collected at indicated time points, allowed to clot for 2 h at room temperature and then centrifuged for 15 min at 1,500 g . Serum samples were stored at −20 °C before analysis. Mortality was recorded for up to 2–3 weeks after the onset of lethal endotoxemia or sepsis to ensure that no additional late deaths occurred. Cytokine measurements Commercially available enzyme-linked immunosorbant assay (ELISA) kits were used to measure the concentrations of HMGB1 (Shino Test Corporation, Tokyo, Japan, ST51011), IL-1β (R&D Systems, MLB00C) and TNF-α (R&D Systems, MTA00B) in serum or the culture medium according to the manufacturer’s instructions. Activity assay Lactate in serum or the culture medium was measured with colorimetric L -Lactate Assay Kit (Abcam, Cambridge, MA, USA, ab65331) according to the manufacturer’s instructions. HDAC activity was measured with the fluorometric HDAC Activity Assay kit (Abcam, ab156064) according to the manufacturer’s instructions. HIF1α DNA binding activity in nuclear extracts was measured with HIF1α Transcription Factor Assay Kit (Cayman, Ann Arbor, MI, USA, 10006910) according to the manufacturer’s instructions. PKM2 activity was measured by a lactate dehydrogenase-coupled enzyme assay [27] , [60] . The assay was carried out with 1 μg of cell lysates with an enzyme buffer (50 mM Tris-HCl (pH 7.5), 100 mM KCl, 10 mM MgCl 2 , 0.9 mM adenosine diphosphate, 0.6 mM PEP, 0.12 mM β-nicotinamide adenine dinucleotide and 4.8 U ml −1 lactate dehydrogenase). Enzyme activity can be measured at 340 nm absorbance by spectrophotometry. RNA interference All shRNA constructs were in the pLKO.1 backbone (Sigma). Transfection with indicated shRNA ( Supplementary Table 1 ) and control empty shRNA (SHC001) from Sigma were performed using FuGENE HD Transfection Reagent (Roche Applied Science) or MISSION shRNA Lentiviral Transduction (Sigma) according to the manufacturer’s instructions. Western blot analysis After extraction, proteins in cell lysates were first resolved by SDS–PAGE, and then transferred to nitrocellulose membrane and subsequently incubated with the primary antibody. The antibodies to HMGB1 (ab18256; 1:1,000) and HIF1α (ab16066; 1:1,000) were obtained from Abcam. The antibodies to PKM1 (7067; 1:1,000), PKM2 (4053; 1:1,000), acetylated-lysine (9441; 1:1,000) and actin (3700; 1:1,000) were obtained from Cell Signaling Technology (Danvers, MA, USA). The antibody to GPR81 (SAB1300089; 1:200) was obtained from Sigma. After incubation with peroxidase-conjugated secondary antibodies, the signals were visualized by enhanced chemiluminescence (Pierce, Rockford, IL, USA, 32106) according to the manufacturer’s instruction. The relative band intensity was quantified using the Gel-pro Analyzer software (Media Cybernetics, Bethesda, MD, USA). Quantitative real-time PCR Total RNA was extracted using TRI reagent (Sigma) according to the manufacturer’s instructions. First-strand complementary DNA was synthesized from 1 μg of RNA using the iScript cDNA Synthesis kit (Bio-Rad, Hercules, CA). cDNA from various cell samples were amplified by real-time quantitative PCR with specific primers ( Supplementary Table 2 ). Immunoprecipitation analysis Cells were lysed at 4 °C in RIPA buffer (Millipore). Before immunoprecipitation, samples containing equal amounts of proteins were pre-cleared with Protein A sepharose (Millipore) and subsequently incubated with various irrelevant IgG or specific antibodies (PKM2 (4053; 2 μg ml −1 ) and HMGB1 (ab18256; 2 μg ml −1 )] in the presence of protein A sepharose beads. The beads were washed three times with RIPA buffer and the immune complexes were eluted from the beads and subjected to SDS–PAGE and immunoblot analysis as previously described [61] , [62] . Oxidative phosphorylation and glycolysis assay Cellular OXPHOS and glycolysis were monitored using the Seahorse Bioscience Extracellular Flux Analyzer (XF24, Seahorse Bioscience Inc., North Billerica, MA, USA) by measuring the OCR (indicative of respiration) and ECAR (indicative of glycolysis) [63] , [64] . Briefly, 30,000–50,000 cells were seeded in 24-well plates designed for XF24 in 150 μl of appropriate growth media and incubated overnight. Before measurements, cells were washed with unbuffered media once, then immersed in 675 μl unbuffered media and incubated in the absence of CO 2 for 1 h. OCR and ECAR were then measured in a typical 8-min cycle of mix (2–4 min), dwell (2 min) and measure (2–4 min) as recommended by Seahorse Bioscience. Statistical analysis Data are expressed as means±s.e.m. of two or three independent experiments. Significance of differences between groups was determined by analysis of variance LSD test. The Kaplan–Meier method was used to compare the differences in mortality rates between groups. A P -value<0.05 was considered statistically significant. How to cite this article: Yang, L. et al . PKM2 regulates the Warburg effect and promotes HMGB1 release in sepsis. Nat. Commun. 5:4436 doi: 10.1038/ncomms5436 (2014).